Neurodegeneration inC. elegansmodels of ALS requires TIR-1/Sarm1 immune pathway activation in neurons Amyotrophic lateral sclerosis (ALS) is a neurodegenerative disease thought to employ cell non-autonomous mechanisms where neuronal injury engages immune responses to influence disease progression. Here we show that the expression of mutant proteins causative for ALS in Caenorhabditis elegans motor neurons induces an innate immune response via TIR-1/Sarm1. Loss of function mutations in tir-1 , associated downstream kinases, and the transcription factor atf-7 all suppress motor neuron degeneration. The neurosecretory proteins UNC-13 and UNC-31 are required for induction of the immune response as well as the degeneration of motor neurons. The human orthologue of UNC-13, UNC13A, has been identified as a genetic modifier of survival in ALS, and we provide functional evidence of UNC-13/UNC13A in regulating motor neuron degeneration. We propose that the innate immune system reacts to the presence of mutant proteins as a contagion, recruiting a pathogen resistance response that is ultimately harmful and drives progressive neurodegeneration. Amyotrophic lateral sclerosis (ALS) is a fatal neurodegenerative disease characterized by a progressive and selective loss of motor neurons in the brain and spinal cord [1] . At the cellular and molecular levels, numerous mechanisms have been associated with ALS including impaired axonal transport, mitochondrial dysfunction, pathological induction of the integrated stress response and neuroinflammation [2] . Over two-dozen genes are associated with ALS, including genes encoding the DNA/RNA-binding proteins TAR DNA Binding Protein 43 (TDP-43) and fused in sarcoma (FUS) [3] . A great challenge remains in functionally linking these ALS mutations to pathogenic mechanisms, and with the recent discovery of so many new genes comes the need to develop experimentally tractable models [4] . As many genes linked to ALS are evolutionarily conserved, we turned to the nematode Caenorhaditis elegans to develop in vivo models of TDP-43 and FUS motor neuron degeneration [5] . We have used these C. elegans ALS models to investigate cellular mechanisms underlying motor neuron degeneration [6] , [7] , [8] , as well as for drug discovery [9] , [10] , [11] . Given the importance of neuroinflammation to the pathological progression of neurodegeneration, including for ALS [12] , we set out to investigate fundamental immune response signalling in our ALS models. C. elegans possesses an innate immune system that is induced in response to viral or microbial infection [13] . One antimicrobial defence pathway in C. elegans consists of tir-1 , encoding a Toll Interleukin 1 Receptor (TIR) domain adaptor protein, which is orthologous to human Sarm1 (sterile alpha and armadillo repeats) [14] , as well as the downstream kinases NSY-1, SEK-1 and PMK-1 (ref. 15 ). Microbial infection triggers this signalling pathway to activate the transcription factor ATF-7, leading to increased transcription of numerous genes including one encoding the antimicrobial peptide NLP-29 (ref. 16 ) (neuropeptide-like protein 29). C. elegans is an established model for investigating conserved genetic pathways that regulate the cellular stress response and neurodegeneration [4] . In this study, using transgenic C. elegans models for ALS we investigate the role of the innate immune response and discover that the TIR-1 pathway regulates motor neuron degeneration caused by mutant TDP-43 and FUS proteins. Mutant ALS proteins activate an innate immune response We created C. elegans strains expressing full-length, untagged, human TDP-43 or FUS proteins in motor neurons. Transgenic C. elegans expressing mutant TDP-43 or FUS in their motor neurons show age-dependent motility defects leading to paralysis and motor neuron degeneration at a rate significantly higher than wild-type TDP-43 or FUS control strains [5] . These behavioural and degenerative phenotypes typically develop over 7–12 days of adulthood for worms cultured on petri plates. To investigate whether mutant TDP-43 or FUS proteins engaged the innate immune response, we crossed our transgenic ALS models with a transgenic strain expressing the reporter nlp-29::GFP. nlp-29 encodes an antimicrobial, neuropeptide-like protein that is expressed in hypodermal and intestinal tissue ( Supplementary Fig. 1 ) following fungal infection, physical injury or osmotic stress [17] . Thus, the nlp-29::GFP reporter brightly fluoresces when the animal is subjected to infectious and/or wounding conditions [18] , [19] . At day 9 of adulthood we observed that mutant TDP-43 A315T or FUS S57Δ transgenics, but not wild type TDP-43 or FUS control strains, caused a significant increase in nlp-29::GFP expression ( Fig. 1a–d ). 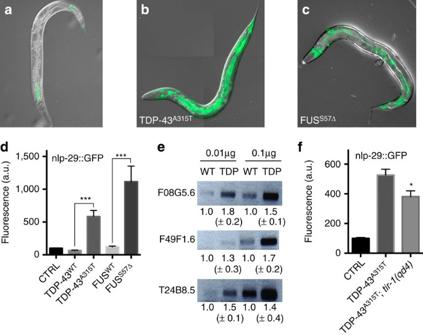Figure 1: Activation of immune-linked gene transcription in TDP-43 and FUS ALS models. (a–c) nlp-29::GFP reporter expression in intestinal and hypodermal tissue from (a) control, (b) TDP-43A315Tand (c) FUSS57Δanimals. (d) Quantification of nlp-29::GFP fluorescence in control animals (CTRL,n=78) compared with animals also expressing TDP-43WT(n=36), TDP-43A315T(n=36), FUSWT(n=26), FUSS57Δ(n=72). Error bars represent s.e.m., ***P<0.001, two-tailedt-test. (e) Semi-quantitative RT-PCR of three immune response genes in mutant TDP-43 transgenics (TDP) versus wild-type controls. Shown are representative images, and the data are the mean±s.e.m. of three independent experiments normalized to control samples. (f) Quantification of nlp-29::GFP fluorescence TDP-43A315T;tir-1(qd4)animals (n=15) versus controls (CTRL,n=21; TDP-43A315T,n=18). *P<0.05, two-tailedt-test. Figure 1: Activation of immune-linked gene transcription in TDP-43 and FUS ALS models. ( a – c ) nlp-29::GFP reporter expression in intestinal and hypodermal tissue from ( a ) control, ( b ) TDP-43 A315T and ( c ) FUS S57Δ animals. ( d ) Quantification of nlp-29::GFP fluorescence in control animals (CTRL, n =78) compared with animals also expressing TDP-43 WT ( n =36), TDP-43 A315T ( n =36), FUS WT ( n =26), FUS S57Δ ( n =72). Error bars represent s.e.m., *** P <0.001, two-tailed t -test. ( e ) Semi-quantitative RT-PCR of three immune response genes in mutant TDP-43 transgenics (TDP) versus wild-type controls. Shown are representative images, and the data are the mean±s.e.m. of three independent experiments normalized to control samples. ( f ) Quantification of nlp-29::GFP fluorescence TDP-43 A315T ; tir-1(qd4) animals ( n =15) versus controls (CTRL, n =21; TDP-43 A315T , n =18). * P <0.05, two-tailed t -test. Full size image We extended our investigation of innate immune response signalling by examining the expression of several additional genes. The genes F08G5.6 , F49F1.6 and T24B8.5 function within the tir-1 pathway and show increased expression under infection conditions [20] , [21] . We observed increased expression of these genes in animals expressing mutant TDP-43 proteins compared with controls ( Fig. 1e ). These data demonstrate that the expression of mutant ALS proteins in motor neurons induces the expression of genes associated with the innate immune response in vivo . As tir-1 is required for the induction of nlp-29 expression during infection [16] , we wondered whether tir-1 was also required for nlp-29::GFP expression by mutant ALS proteins. Using the null mutation tir-1(qd4) we constructed a TDP-43 A315T ; nlp-29p::GFP ; tir-1(qd4) strain and observed it had less fluorescence compared with a TDP-43 A315T ; nlp-29::GFP strain ( Fig. 1f ), suggesting the induction of the immune response by mutant proteins partially requires the tir-1 pathway. Next, we wondered whether the induction of nlp-29::GFP was specific to TDP-43 or FUS, or perhaps could be triggered by other misfolded proteins. We created strains to model polyglutamine toxicity by expressing mutant human ATXN3 in the worm’s motor neurons. Machado-Joseph disease is caused by a trinucleotide CAG repeat expansion (coding for glutamine) in ATXN3 (ref. 22 ). We created strains expressing human ataxin-3 with either 14 polyglutamine repeats (wild-type allele) or 89 polyglutamine repeats (disease allele). These same mutant polyQ89 ataxin-3 proteins have been previously shown to misfold and cause neurodegeneration in cell culture and Drosophila models [23] . These ataxin-3 C. elegans strains were then crossed with the nlp-29::GFP reporter and we observed that the polyQ14 or polyQ89 transgenes did not induce nlp-29::GFP expression ( Supplementary Fig. 2 ). These data demonstrate that ALS-associated mutations in TDP-43 and FUS specifically induce nlp-29::GFP expression, suggesting they employ pathogenic mechanisms distinct from polyglutamine toxicity. The endoplasmic reticulum (ER) stress response and increased levels of oxidative stress are associated with the expression of mutant TDP-43 or FUS proteins in cells [24] . Thus, we investigated whether nlp-29::GFP expression was induced by either ER or oxidative stress. Chemical induction of the ER stress response by tunicamycin, or the in vivo production of oxidative stress by juglone did not activate nlp-29::GFP expression ( Supplementary Fig. 3a,b ). Finally, the antioxidant n-acetylcysteine did not extinguish fluorescence signals in TDP-43 A315T ; nlp-29::GFP animals, suggesting that oxidative stress does not play a role in inducing nlp-29::GFP expression ( Supplementary Fig. 3c ). Induction of an innate immune response requires neurosecretion In our C. elegans models, the expression of mutant TDP-43 or FUS proteins is limited to 26 GABAergic neurons [5] , yet the nlp-29::GFP reporter shows expression in the intestine and hypodermis ( Supplementary Fig. 1 ). These observations suggest some sort of cellular communication event occurs between the motor neurons and distal tissues like the intestine and hypodermis. There are numerous developmental and behavioural phenomena that rely on communication between the nervous system and intestinal tissue in C. elegans . For example, neuron-intestine communication via insulin-like peptides regulates the dauer diapause decision during development [25] , and intestinal signalling to GABAergic neurons regulates a highly coordinated defecation motor programme [26] . Furthermore, we previously reported a cell-nonautonomous effect for mutant TDP-43 proteins in activating the ER unfolded protein response. hsp-4 encodes a C. elegans Hsp70 protein orthologous to mammalian Grp78/BiP, and the transgenic C. elegans hsp-4::GFP reporter is activated in intestinal tissue by the expression of mutant TDP-43 in motor neurons [6] . The relentless disease progression seen in ALS may be due to extracellular mechanisms including the activity of unknown secreted molecules capable of spreading disease to adjacent tissues [27] . Recent reports show that the cell non-autonomous activation of the ER stress [28] and heat-shock [29] responses in C. elegans requires proteins responsible for neurosecretion, namely small clear vesicles (SCV) releasing neurotransmitters, and dense core vesicles (DCV) that release neuropeptides [30] , [31] . Thus, we wondered whether the mutant TDP-43 A315T mediated activation of nlp-29::GFP was dependent on neurosecretion. unc-13 encodes a synaptic protein essential for the release of SCV, while unc-31 encodes a calcium-dependent activator protein required for the release of DCV [30] , [31] . Using loss of function mutations for unc-13 and unc-31 , we created TDP-43 A315T ; nlp-29::GFP; unc-13(e540) and TDP-43 A315T ; nlp-29::GFP; unc-31(e928) strains and observed that these animals had significantly less fluorescence than TDP-43 A315T ; nlp-29::GFP controls ( Fig. 2a–c ). 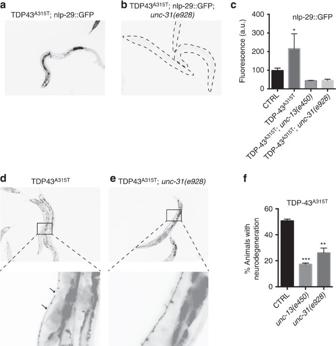Figure 2: Induction of the innate immune response and neurodegeneration requireunc-13andunc-31. Representative images of nlp-29::GFP expression in (a) TDP-43A315Tand (b) TDP-43A315T;unc-31(e928)animals. (c) Quantification of nlp-29::GFP fluorescence in TDP-43A315T;unc-13(e450)(n=37), and TDP-43A315T;unc-31(e928)(n=38) animals plus controls (CTRL,n=45; TDP-43A315T,n=57). *P<0.05, two-tailedt-test, error bars represent s.e.m. Representative images of (d) TDP-43A315Tand (e) TDP-43A315T;unc-31(e928)animals expressing the unc-47::GFP reporter that fluoresces in GABAergic motor neurons. Degeneration, observed as gaps or breaks along neuronal processes, is indicated (arrows). (f) Quantification of motor neuron degeneration in TDP-43A315T;unc-13(e450)and TDP-43A315T;unc-31(e928)animals versus TDP-43A315Tcontrols **P<0.01, ***P<0.001, two-tailedt-test, error bars represent s.e.m. The fluorescent GFP images have been transformed to black and white and photo-reversed. Figure 2: Induction of the innate immune response and neurodegeneration require unc-13 and unc-31 . Representative images of nlp-29::GFP expression in ( a ) TDP-43 A315T and ( b ) TDP-43 A315T ; unc-31(e928) animals. ( c ) Quantification of nlp-29::GFP fluorescence in TDP-43 A315T ; unc-13(e450) ( n =37), and TDP-43 A315T ; unc-31(e928) ( n =38) animals plus controls (CTRL, n =45; TDP-43 A315T , n =57). * P <0.05, two-tailed t -test, error bars represent s.e.m. Representative images of ( d ) TDP-43 A315T and ( e ) TDP-43 A315T ; unc-31(e928) animals expressing the unc-47::GFP reporter that fluoresces in GABAergic motor neurons. Degeneration, observed as gaps or breaks along neuronal processes, is indicated (arrows). ( f ) Quantification of motor neuron degeneration in TDP-43 A315T ; unc-13(e450) and TDP-43 A315T ; unc-31(e928) animals versus TDP-43 A315T controls ** P <0.01, *** P <0.001, two-tailed t -test, error bars represent s.e.m. The fluorescent GFP images have been transformed to black and white and photo-reversed. Full size image Of interest, UNC13A is the human orthologue of C. elegans unc-13 , and UNC13A has recently been identified as a modifier disease progression in ALS patients [32] , [33] , [34] . Thus, we hypothesized that signalling from the motor neurons via unc-13 and unc-31 may affect the toxicity of mutant ALS proteins. As unc-13 and unc-31 mutants show strong defects in motility, we were unable to test whether they affected the age-dependent paralysis phenotype displayed by mutant TDP-43 A315T animals. Instead we examined whether blocking neurosecretion by unc-13 or unc-31 would have an effect on neurodegeneration. Animals expressing mutant TDP-43 proteins show age-dependent degeneration of motor neurons [5] . Examination of the TDP-43 A315T ; unc-13(e540) and TDP-43 A315T ; unc-31(e928) strains revealed significantly decreased motor neuron degeneration compared with TDP-43 A315T alone ( Fig. 2d–f ). These data suggest that neurosecretion is required for activation of the innate immune response, as well as neurodegeneration elicited by mutant ALS proteins. Furthermore, our data support the notion that UNC-13/UNC13A is a functional modifier of ALS disease progression. TIR-1 is required for motor neuron degeneration We next set out to determine whether the tir-1 pathway actively contributes to neuronal dysfunction and neurodegeneration in our ALS models. We constructed strains with a loss of function mutation for tir-1 along with transgenics expressing mutant TDP-43 or FUS proteins. As described above, transgenic worms expressing mutant TDP-43 or FUS proteins show age-dependent motility defects leading to progressive paralysis and the degeneration of motor neurons [5] . We observed that TDP-43 A315T ; tir-1(qd4) and FUS S57Δ ; tir-1(qd4) animals had significantly lower rates of paralysis compared with TDP-43 A315T or FUS S57Δ alone with no effects on transgene expression ( Fig. 3a–d ). We also observed suppression of motor neuron degeneration in TDP-43 A315T ; tir-1(qd4) and FUS S57Δ ; tir-1(qd4) animals compared with control strains ( Fig. 3e ). 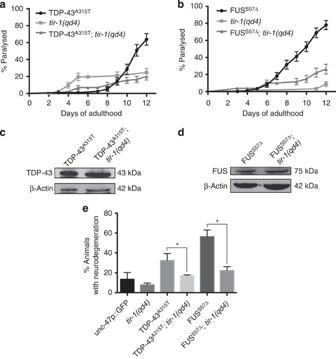Figure 3:tir-1promotes TDP-43A315Tor FUSS57Δ-induced paralysis and neurodegeneration. The loss of function mutationtir-1(qd4)suppressed motility defects and progressive paralysis induced by (a) TDP-43A315T(TDP-43A315T,n=211;tir-1(qd4),n=229; TDP-43A315T;tir-1(qd4),n=187) or (b) FUSS57Δ(FUSS57Δ,n=159;tir-1(qd4),n=151; FUSS57Δ,tir-1(qd4),n=163) compared with controls,P<0.001, Log-rank (Mantel-Cox)-test, error bars represent s.e.m. Expression of (c) TDP-43 or (d) FUS proteins measured by western blot. (e) Quantification of neurodegeneration in GABAergic motor neurons observed in TDP-43A315Tor FUSS57Δtransgenics with and without thetir-1(qd4)mutation, *P<0.05, two-tailedt-test, error bars represent s.e.m. Figure 3: tir-1 promotes TDP-43 A315T or FUS S57Δ -induced paralysis and neurodegeneration. The loss of function mutation tir-1(qd4) suppressed motility defects and progressive paralysis induced by ( a ) TDP-43 A315T (TDP-43 A315T , n =211; tir-1(qd4) , n =229; TDP-43 A315T ; tir-1(qd4) , n =187) or ( b ) FUS S57Δ (FUS S57Δ , n =159; tir-1(qd4) , n =151; FUS S57Δ , tir-1(qd4) , n =163) compared with controls, P <0.001, Log-rank (Mantel-Cox)-test, error bars represent s.e.m. Expression of ( c ) TDP-43 or ( d ) FUS proteins measured by western blot. ( e ) Quantification of neurodegeneration in GABAergic motor neurons observed in TDP-43 A315T or FUS S57Δ transgenics with and without the tir-1(qd4) mutation, * P <0.05, two-tailed t -test, error bars represent s.e.m. Full size image In laboratory settings, bacteria are the primary food source for C. elegans [35] . As the tir-1 pathway can initiate an immune response due to bacterial infection, we wished to determine the contribution of any bacterial influence on the suppression of TDP-43 motor neuron toxicity by examining the rate of paralysis of TDP-43 A315T ; tir-1(qd4) animals grown on heat-killed OP50 bacteria. We observed suppression of TDP-43 A315T mediated paralysis similar to animals grown on live bacteria ( Supplementary Fig. 4 ), suggesting that the presence of the bacterial food source does not influence tir-1 or TDP-43 motor neuron phenotypes. In addition, we confirmed that tir-1(qd4) suppressed motility defects using an automated assay that measures the movement of C. elegans grown in liquid culture ( Supplementary Fig. 5 ). These data suggest that tir-1 contributes to neuronal dysfunction and degeneration caused by ALS-associated mutant proteins. TIR-1 activity in the nervous system promotes degeneration Our data thus far indicate that mutant ALS proteins induce the expression of immune response genes via the tir-1 pathway, and that blocking tir-1 suppresses motor neuron degeneration caused by mutant ALS proteins. Next we asked whether tir-1 activity in the nervous system, distal tissues, or both was required for the paralysis phenotype caused by mutant TDP-43 proteins. To answer these questions we turned to an RNA-interference (RNAi) approach allowing for tissue-specific inhibition of tir-1 activity. We created transgenic lines expressing mutant TDP-43 in conjunction with C. elegans strains that were sensitive to RNAi only within neurons, body wall muscle cells or intestinal tissue [8] . We observed that tir-1 (RNAi) suppressed paralysis in worms sensitized to RNAi in the nervous system, but failed to suppress paralysis in strains sensitized to RNAi in body wall muscle cells or intestinal tissue ( Supplementary Fig. 6 ). These data suggest that activation of the tir-1 signalling pathway within the nervous system is required for mutant TDP-43 toxicity. Our emerging model is that mutant ALS proteins in the nervous system initiate a neurosecretory event that triggers an immune response in distal tissues (intestine, hypodermis) as well as locally in motor neurons leading to neurodegeneration. TIR-1 pathway kinases promote neurodegeneration Essential to the TIR-1 mediated response is a signalling cascade involving the kinases NSY-1/MAP3K, SEK-1/MAPK and PMK-1/p38 MAPK. To determine whether this signalling cassette is essential for motor neuron dysfunction and degeneration, we crossed the TDP-43 A315T transgenics with loss of function mutations for nsy-1 , sek-1 or pmk-1 . We observed significant reduction of TDP-43 A315T induced paralysis and neurodegeneration in TDP-43 A315T ; nsy-1(ok593) , TDP-43 A315T ; sek-1(km4) , and TDP-43 A315T ; pmk-1(km25) compared with TDP-43 A315T control strains ( Fig. 4a,b ). 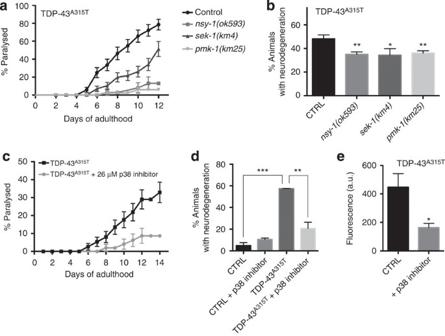Figure 4: Inhibition of the TIR-1 pathway kinase signalling pathway suppresses motor neuron degeneration. Loss of function mutationsnsy-1(ok593)(n=64),sek-1(km4)(n=112) orpmk-1(km25)(n=142) suppressed (a) TDP-43A315T-mediated paralysis compared with TDP-43A315Talone (n=154), (P<0.001) and (b) motor neuron degeneration (*P<0.05, **P<0.01). The p38 kinase inhibitor SB203580 suppressed TDP-43A315T-induced (c) paralysis (P<0.001, control,n=181;+p38 inhibitor,n=144), (d) neurodegeneration and (e) nlp-29::GFP expression versus untreated controls (CTRL,n=20; p38 inhibitor,n=15). Log-rank (Mantel-Cox)-test for paralysis assays, two-tailedt-test for all other experiments. *P<0.05, **P<0.01, ***P<0.001. Error bars represent s.e.m. Figure 4: Inhibition of the TIR-1 pathway kinase signalling pathway suppresses motor neuron degeneration. Loss of function mutations nsy-1(ok593) ( n =64), sek-1(km4) ( n =112) or pmk-1(km25) ( n =142) suppressed ( a ) TDP-43 A315T -mediated paralysis compared with TDP-43 A315T alone ( n =154), ( P <0.001) and ( b ) motor neuron degeneration (* P <0.05, ** P <0.01). The p38 kinase inhibitor SB203580 suppressed TDP-43 A315T -induced ( c ) paralysis ( P <0.001, control, n =181;+p38 inhibitor, n =144), ( d ) neurodegeneration and ( e ) nlp-29::GFP expression versus untreated controls (CTRL, n =20; p38 inhibitor, n =15). Log-rank (Mantel-Cox)-test for paralysis assays, two-tailed t -test for all other experiments. * P <0.05, ** P <0.01, *** P <0.001. Error bars represent s.e.m. Full size image As genetic loss-of-function mutations in genes encoding the kinases NSY-1, SEK-1 and PMK-1 all suppressed TDP-43 motor neuron toxicity, we hypothesized that these proteins would be excellent targets for inhibition of their activity by small molecules. Furthermore, mitogen-activated protein kinases have been extensively studied for pharmacological targeting of the innate immune response [36] , and some of these small molecules are clinically approved. We tested the p38 kinase inhibitor SB203580 and observed that it reduced paralysis and neurodegeneration in TDP-43 A315T transgenics ( Fig. 4c,d ). Finally, we treated TDP-43 A315T ; nlp-29::GFP animals with SB203580 and observed decreased fluorescence compared with untreated controls ( Fig. 4e ), suggesting that chemically inhibiting PMK-1 leads to a concomitant reduction of the innate immune response triggered by mutant ALS proteins. Thus, our data demonstrate that inhibition of the kinase signalling cascade pathway downstream from TIR-1 reduces mutant TDP-43-dependent immune system activation and motor neuron degeneration. Motor neuron degeneration requires ATF-7 Signalling via TIR-1, NSY-1, SEK-1 and PMK-1 requires the activity of the transcription factor ATF-7 to induce the expression of innate immune response genes in response to infection. Thus, we predicted that atf-7 was required for the neurodegeneration caused by the expression of mutant ALS proteins in motor neurons. Using the loss of function mutation atf-7(qd22) we created TDP-43 A315T ; atf-7(qd22) animals and observed that these animals had significant reductions in the rate of paralysis and neurodegeneration compared with TDP-43 A315T controls ( Fig. 5 ). These data are consistent with the notion that that atf-7 functions as a downstream effector of the tir-1 pathway, and that the chronic activation of ATF-7 promotes motor neuron degeneration caused by mutant ALS proteins. 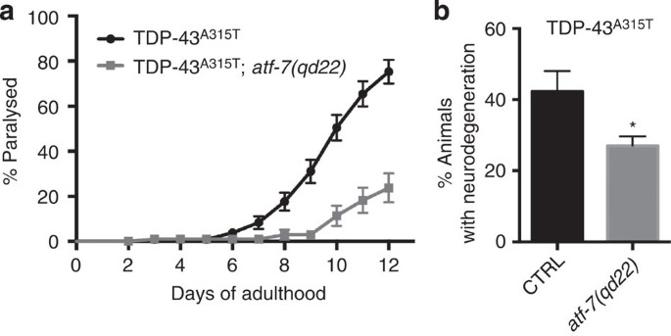Figure 5:atf-7is required for TDP-43 mediated motor neuron degeneration. The loss of function mutationatf-7(qd22)suppresses (a) paralysis (P<0.001, CTRL,n=179;atf-7(qd22),n=198) and (b) motor neuron degeneration (*P<0.01) in transgenic TDP-43A315Tanimals compared with controls. The log-rank (Mantel-Cox)-test was used for paralysis assays and two-tailedt-tests were used for neurodegeneration experiments. Figure 5: atf-7 is required for TDP-43 mediated motor neuron degeneration. The loss of function mutation atf-7(qd22) suppresses ( a ) paralysis ( P <0.001, CTRL, n =179; atf-7(qd22) , n =198) and ( b ) motor neuron degeneration (* P <0.01) in transgenic TDP-43 A315T animals compared with controls. The log-rank (Mantel-Cox)-test was used for paralysis assays and two-tailed t -tests were used for neurodegeneration experiments. Full size image Next we investigated whether or not the tir-1 signalling pathway may generally affect the lifespan of worms, thus perhaps non-specifically delaying the onset of degenerative phenotypes in transgenics expressing mutant ALS proteins. However, lifespan analyses indicated that none of the mutations tested here including for tir-1 , nsy-1 , sek-1 , pmk-1 or atf-7 extended the lifespan of mutant TDP-43 transgenics ( Supplementary Fig. 7 ). Mutant TDP-43 does not confer systemic stress resistance Finally, a recent report demonstrated that DNA damage in C. elegans germ cells provokes a system wide innate immune response conferring systemic stress resistance [37] . Thus, we wondered whether mutant ALS proteins in the nervous system would likewise induce stress resistance. However, we previously reported that TDP-43 A315T transgenics have normal lifespan [5] , and here we observed that they displayed normal resistance to osmotic or thermal stress, but were sensitive to oxidative stress ( Supplementary Fig. 8 ). Thus, the expression of mutant TDP-43 proteins in motor neurons does not produce a general stress resistance phenotype, suggesting that neuronal proteotoxicty may elicit a stress response distinct from DNA damage in the germline. DCAR-1 is not involved in motor neuron degeneration TIR-1 is an adaptor protein believed to mediate signalling downstream from an otherwise unknown cell surface receptor proteins. Recently, the dihydrocaffeic acid receptor DCAR-1 was identified as a component of the TIR-1 signalling pathway in response to epidermal infection [38] . We wondered whether DCAR-1 also contributed to neurodegeneration from mutant ALS proteins, but found that dcar-1 null mutations failed to suppress mutant TDP-43-mediated paralysis and motor neuron degeneration ( Supplementary Fig. 9 ). Thus, additional upstream receptor proteins may be involved in transmitting signals in response to neuronal injury via TIR-1, but distinct from the DCAR-1 pathway. In higher systems, a variety of immune and non-immune cell types express toll-like receptors on their cell surface that recognize microbial pathogen-associated molecular patterns (PAMPs) and other receptors that recognize tissue damage signals, such as alarmins. Alarmins are often small molecules that are released into the extracellular environment by damaged or dying cells. C. elegans maintains extensive surveillance pathways to monitor fundamental cellular activities, that when disrupted are interpreted as attack by pathogens [39] . TDP-43 and FUS both contain low-complexity prion-like domains [40] , and TDP-43 has been reported to propagate between cells by an exosome-mediated mechanism [41] . Thus, it is possible that mutant TDP-43 or FUS could engage the innate immune response, either directly or in response to alarmins released by damaged neurons. In this context, mutant ALS proteins in neurons may elicit an immune response as part of a host defense reaction against pathogens, or to aid tissue repair, or both. Future unbiased molecular and genetic analyses exploiting the power of the C. elegans system may help identify the molecules necessary to induce the expression of nlp-29::GFP. Nonetheless, chronic engagement of the TIR-1 pathway in motor neurons ultimately leads to neurodegeneration ( Fig. 6 ). 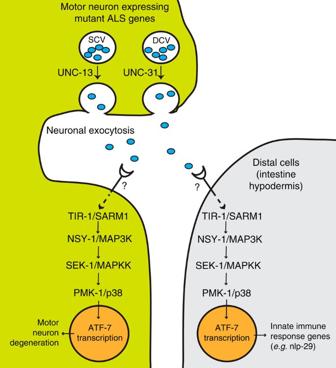Figure 6: Motor neuron degeneration via the TIR-1 signalling pathway. Motor neurons expressing mutant ALS genes promote the release of a signalling molecule via neuronal exocytosis. UNC-13 is required for the release of small clear vesicles (SCV) and neurotransmitters, while UNC-31 is required for the release of dense core vesicles (DCV) containing mainly neuropeptides. The unknown secreted molecules then activate the TIR-1 signalling pathway resulting in the increased transcription of immune response genes, likenlp-29in distal intestinal and hypodermal cells. At the same time the secreted molecules activate the TIR-1 pathway in motor neurons leading to neurodegeneration. Figure 6: Motor neuron degeneration via the TIR-1 signalling pathway. Motor neurons expressing mutant ALS genes promote the release of a signalling molecule via neuronal exocytosis. UNC-13 is required for the release of small clear vesicles (SCV) and neurotransmitters, while UNC-31 is required for the release of dense core vesicles (DCV) containing mainly neuropeptides. The unknown secreted molecules then activate the TIR-1 signalling pathway resulting in the increased transcription of immune response genes, like nlp-29 in distal intestinal and hypodermal cells. At the same time the secreted molecules activate the TIR-1 pathway in motor neurons leading to neurodegeneration. Full size image We investigated TIR-1 as a modifier of TDP-43 and FUS proteotoxicity due to its role in the C. elegans innate immune system. The Drosophila orthologue, dSarm, was identified from a forward genetic screen for mutations that promoted long-term survival of severed axons, and this protective activity was also observed in mice with a knockout allele for Sarm1 [42] , [43] . These data suggest that TIR-1/Sarm1 may actively participate in a cell death programme targeting damaged axons, which may be relevant to the axon ‘dying back’ phenotype observed in neurodegenerative diseases including ALS [44] . Furthermore, tir-1 has been linked to a non-apoptotic cell death pathway supporting our observations about ced-3 /Caspase-3-independent mechanisms regulating TDP-43 toxicity in our C. elegans ALS models [8] . We recently reported that motor neuron degeneration caused by mutant TDP-43 proceeds through dysregulated intracellular calcium signalling resulting in a necrosis-like degenerative phenotype [8] . Here, an accumulation of cytosolic calcium activates calpain proteases that in turn activate killer aspartyl proteases leading to cell destruction [45] . A recent study using mammalian models demonstrated that axonal injury phenotypes mediated by Sarm1 also require calpain proteases [46] . Thus, there may be a convergence of the TIR-1/Sarm1 pathway in regulating motor neuron degeneration via calpain proteases in ALS. A cardinal feature of many late-onset neurodegenerative diseases is the accumulation of misfolded proteins suggesting that there may be common pathogenic mechanisms underlying many of these diseases. Our data suggest that the pathogenic mechanisms of TDP-43 and FUS are similar in their ability to provoke an innate immune response, and this is distinct from other forms of proteotoxicity, namely polyglutamine toxicity in this instance. At this point we do not know whether the RNA homeostasis functions of TDP-43 and FUS are implicated in activation of the tir-1 pathway and the innate immune response, or whether this extends to all genes associated with ALS. The development of new ALS models will help answer this question. Essential to neurodegeneration and activation of nlp-29::GFP by mutant ALS proteins are the genes unc-13 and unc-31 , which encode proteins with roles in exocytosis [31] . SCV generally contain classical neurotransmitters, while DCV mainly transport neuropeptides, thus it is not clear what, if any, cargos are shared between the two to induce the expression of nlp-29::GFP in our ALS models. However, there are similarities between SCV and DCV exocytosis; thus, there may be a common mechanism, or secreted molecule, signalling from diseased motor neurons. The C. elegans unc-13 gene encodes a presynaptic protein involved in the release of synaptic vesicles [30] . unc-13 is evolutionarily conserved and the human orthologue UNC13A also has roles in the regulation of neurotransmitter release at neuromuscular junctions [47] . Directly relevant to ALS, several research groups have uncovered UNC13A as a potential susceptibility gene for ALS [32] , [33] , [34] , [48] . Thus, UNC13A may be a modifier of disease survival and could be a target for therapeutic development. We observed that deletion of unc-13 suppressed motor neuron degeneration caused by mutant TDP-43 proteins. Thus, we provide the first functional validation of unc-13/UNC13A as a modifier of motor neuron degeneration caused by mutant ALS proteins. TIR-1 is believed to act as adaptor protein downstream from the G protein-coupled receptor DCAR-1 (ref. 38 ), but we observed that genetic ablation of dcar-1 did not rescue motility defects or neurodegeneration phenotypes caused by mutant TDP-43. These data suggest that other receptor proteins may be responsible for modulating neuronal degeneration in conjunction with TIR-1. Recent work has demonstrated interactions between the SAM (sterile α motif) and TIR domains in Sarm1 are responsible for axonal degeneration phenotypes [43] , suggesting that inhibiting these domains may be a therapeutic strategy for limiting neurodegeneration. However, the kinases downstream from TIR/Sarm1, including the MAPK p38, have been the subject of numerous studies and many small molecule inhibitors of these protein kinases have been tested including in human clinical trials, most notably for rheumatoid arthritis [49] . Our C. elegans data demonstrate that genetic inhibition of the downstream MAPK pathway suppresses neurodegeneration; thus, these proteins may be excellent targets for inhibition by small molecules. Furthermore, there are a number of FDA approved compounds targeting the MAPK pathway that may have clinical relevance for ALS patients. In summary, we have identified an evolutionarily conserved signalling pathway centred on TIR-1/Sarm1 that regulates motor neuron degeneration caused by mutant TDP-43 and FUS proteins. The components of this pathway regulate the innate immune response and neuronal survival thus providing new targets to aid the development of therapeutic approaches for ALS. Standard methods of culturing and handling C. elegans were followed [35] . Worms were maintained on standard NGM plates streaked with OP50 E. coli . Strains used in this study were obtained from the C. elegans Genetics Center (University of Minnesota, Minneapolis) unless indicated. Strains used in this study include: atf-7(qd22) , dcar-1(tm2484) , frIs7 [ nlp-29 p::GFP, col-12 p::DsRed], nsy-1(ok593) , oxIs12[ unc-47p ::GFP+ lin-15 ], pmk-1(km25) , sek-1(ag1) , tir-1(qd4 ), unc-13(e450) and unc-31(e928) . Mutant strains were outcrossed 4–6 times to N2 before use. Transgenic lines expressing mutant TDP-43 A315T , wild-type TDP-43 (TDP-43 WT ), mutant FUS S57Δ and wild-type FUS (FUS WT ) were previously described [5] and created as follows: Human cDNAs for the TDP-43 and FUS alleles (kind gift from Dr Guy Rouleau, McGill University) were amplified by PCR and cloned into the Gateway vector pDONR221 following the manufacturer’s protocol (Invitrogen). Multisite Gateway recombination was performed with the pDONR TDP-43 clones along with clones containing the unc-47 promoter (kind gift from Dr Erik Jorgensen, University of Utah, and Dr Marc Hammarlund, Yale University), the unc-54 3′ UTR plasmid pCM5.37 (Dr Geraldine Seydoux, Johns Hopkins, Addgene plasmid 17253) and the destination vector pCFJ150 (Dr Erik Jorgensen, University of Utah, Addgene plasmid 19329) to create unc-47p::TDP-43 and unc-47p::FUS expression vectors. Transgenic lines were created by microinjection of unc-119(ed3) worms, multiple lines were generated and strains behaving similarly were kept for further analysis. Transgenes were integrated by UV irradiation and lines were outcrossed to wild-type N2 worms five times before use. Several strains showing comparable phenotypes and transgene expression levels were kept and the strains used in this study include xqIs98 [ unc-47 p::FUS S57Δ ; unc-119(+)], xqIs132 [ unc-47 p::TDP-43 WT ; unc-119 (+)], xqIs133 [ unc-47 p::TDP-43 A315T ; unc-119 (+)] and xqIs173 [ unc-47 p::FUS WT ; unc-119 (+)]. Single-copy transgenic lines Wild-type Ataxin-3-Q14, or mutant Ataxin-3-Q89 cDNAs (from Dr Guy Rouleau, McGill University) were cloned as described above using the Gateway cloning system (Invitrogen) to create unc-47p:: Ataxin-3-Q14 and unc-47p::Ataxin-3-Q89 expression vectors. Transgenic lines were created by microinjection of unc-119(ed3) worms and screened for MoSCi transposon-mediated single-copy insertion of the desired transgene. Several lines were isolated for each transgene of interest and those showing similar behavioural, transgene expression levels and molecular profiles were kept for further analysis. The strains used in this study include XQ350 unc-119(ed3) ; ttTi5605mosII; xqIs350 (unc-47p::ATXN3::CAG14; unc-119(+) ), and XQ351 unc-119(ed3) ; ttTi5605mosII; xqIs351 (unc-47p::ATXN3::CAG89; unc-119(+) ). Western blotting Fifteen plates of worms for each strain were collected with M9 buffer and protein extraction was performed with v/v RIPA, sonicated for 5 min, centrifuged at 16,000g and the supernatants were quantified using BCA Protein Assay Kit (Thermo Scientific). Thirty micrograms per well of proteins were loaded in a 10% polyacrylamide gel for 90 min, transferred to nitrocellulose membranes (BioRad) and immunoblotted. Antibodies used: rabbit anti-TDP-43 (1:1,000, Proteintech), rabbit anti-FUS/TLS (1:500, Abcam) and mouse anti-Actin (1:5,000, MP Biomedical). Blots were visualized with peroxidase-conjugated secondary antibodies and ECL western blotting substrate (Thermo Scientific). Ladder used: Precision Plus Protein Kaleidoscope (BioRad). Densitometry was performed with Photoshop (Adobe). The uncropped scans of western blots are included in Supplementary Fig. 10 . RNAi experiments RNA interference (RNAi)-treated strains were fed E. coli (HT115) containing an empty vector or tir-1 (F13B10.1). RNAi clones from the ORFeome RNAi library (Open Biosystems). RNAi experiments were performed at 20 °C. Worms were grown on Nematode Growth Media enriched with 1 mM isopropyl-ß- D -thiogalactopyranoside. All RNAi paralysis tests were performed using a TDP-43 A315T ; unc-47::GFP in conjunction with the appropriate mutation and transgenes for tissue-specific silencing in neurons, intestine or muscle cells based on strains TU3401, VP303 or NR350, respectively. To minimize developmental effects, L4 worms were grown on plates with RNAi bacteria and assayed for paralysis as adults. Worms were transferred every 2 days. Paralysis assays on solid media Worms expressing TDP-43 or FUS 20–30 adult day 1 of adulthood animals were picked to NGM plates and scored daily for movement over 12 days. Animals were counted as paralysed if they failed to move upon prodding with a worm pick. Worms were scored as dead if they failed to move their head after being prodded on the nose and showed no pharyngeal pumping. All experiments were conducted at 20 °C. Some experiments were conducted by dissolving SB203580 (Sigma) into the NGM plates. Paralysis assay in liquid culture Twenty, adult day 4 worms expressing TDP-43 were transferred to M9 buffer and the number of movements were scored using a WMicrotracker (Phylumtech). Experiments were done in triplicate. Neurodegeneration assays For scoring of neuronal processes for gaps or breakage, TDP-43 or FUS transgenic animals were selected at day 9 of adulthood for visualization of motor neurons processes in vivo . Animals were immobilized in M9 with 5 mM levamisole and mounted on slides with 2% agarose pads. GFP was visualized at 505 nm using a Zeiss Axio Imager M2 microscope. The software used was Zen Pro 2012. Hundred worms were scored per condition. The mean and s.e.m. were calculated for each trial and two-tailed t tests were used for statistical analysis. RT-PCR assays RNA samples were obtained from 15 confluent plates of worms, following Trizol (Invitrogen)/chloroform extraction and quantified with a NanoPhotometer (Implen). 0.01 μg or 0.1 μg of RNA are reverse transcribed with QuantiTect (Qiagen). Primers used include F08G5.6 forward, 5′-AGTTCCAGCTATGGTATATGCTC-3′; F08G5.6 reverse, 5′-CAATGGTTCGTGGGCTCCA-3′; F49F1.6 forward, 5′-GTGCCCAAATTATAGCGTTCCA-3′; F49F1.6 reverse, 5′-CTTCCACAAACTCCACAGGT-3′; T24B8.5 forward, 5′-TGTGCTTGTAGCTTACACTGCTT-3′; T24B8.5 reverse, 5′-CATAGTTTGGGCAGAGACCAG-3′. Fluorescence microscopy For visualization of nlp-29::GFP or unc-47::GFP animals, M9 buffer with 5 mM levamisole was used for immobilization. Animals were mounted on slides with 2% agarose pads. Fluorescent expression for quantification was visualized with a Zeiss Axio Imager M2 microscope. Fluorescent expression was visualized with a DIC microscope Carl Zeiss AxioObserver A1. The software used was AxioVs40 4.8.2.0. Fifteen to forty worms 9 days aged were visualized. Image processing and quantification were done with Adobe Photoshop. To compare fluorescence, we calculated the changes in the ratio (size/intensity of fluorescence). Statistics Paralysis curves were generated and compared using the Log-rank (Mantel-Cox) test. Twenty to forty animals were tested per genotype and repeated at least three times. For fluorescence and neurodegeneration test, non-parametric t test was realized. Prism 5 (GraphPad Software) was used for all statistical analyses. How to cite this article: Veriepe, J. et al . Neurodegeneration in C. elegans models of ALS requires TIR-1/Sarm1 immune pathway activation in neurons. Nat. Commun. 6:7319 doi: 10.1038/ncomms8319 (2015).